Influenza neuraminidase operates via a nucleophilic mechanism and can be targeted by covalent inhibitors Development of novel influenza neuraminidase inhibitors is critical for preparedness against influenza outbreaks. Knowledge of the neuraminidase enzymatic mechanism and transition-state analogue, 2-deoxy-2,3-didehydro- N -acetylneuraminic acid, contributed to the development of the first generation anti-neuraminidase drugs, zanamivir and oseltamivir. However, lack of evidence regarding influenza neuraminidase key catalytic residues has limited strategies for novel neuraminidase inhibitor design. Here, we confirm that influenza neuraminidase conserved Tyr406 is the key catalytic residue that may function as a nucleophile; thus, mechanism-based covalent inhibition of influenza neuraminidase was conceived. Crystallographic studies reveal that 2α,3ax-difluoro- N -acetylneuraminic acid forms a covalent bond with influenza neuraminidase Tyr406 and the compound was found to possess potent anti-influenza activity against both influenza A and B viruses. Our results address many unanswered questions about the influenza neuraminidase catalytic mechanism and demonstrate that covalent inhibition of influenza neuraminidase is a promising and novel strategy for the development of next-generation influenza drugs. It has recently been demonstrated that highly pathogenic H5N1 avian influenza can easily adapt to become airborne-transmissible in mammals [1] , [2] , reminding the world about the pandemic potential of avian influenza viruses [3] , [4] . Moreover, only two drugs, zanamivir and oseltamivir, that function as influenza neuraminidase (NA) inhibitors are currently recommended for use worldwide. Therefore, the development of novel influenza drugs is critical for preparedness against possible future influenza epidemics and pandemics. The influenza A virus genome comprises 8 negative strand RNA segments encoding 13 proteins [5] . Two major glycoproteins, hemagglutinin (HA) and NA, as well as the M2 ion channel, are on the surface of the virions and are therefore highly accessible targets for drug development [6] , [7] . Of these three transmembrane proteins, only NA is known to function as an enzyme and is therefore an ideal target for the design of competitive inhibitors that can mimic catalytic transition-state intermediates [8] . Accordingly, influenza NA is currently the most successful drug-target against influenza virus. Besides NA inhibitors, only M2 ion channel inhibitors have been fully developed; however, the influenza M2 inhibitors amantadine and rimantadine are no longer in use due to serious problems with drug resistance [8] . The design of influenza NA inhibitors is regarded a classical example of rational structure-based drug design, but there are currently only two NA inhibitors, oseltamivir and zanamivir, that are approved for use worldwide [8] . Furthermore, oseltamivir resistance was reported to be highly prevalent in seasonal H1N1 isolates from September 2008 to January 2009 [9] , whereas zanamivir is not orally active and has a short duration of action. Two more recently developed NA inhibitors, laninamivir and peramivir, are approved for use in Japan and still under phase III clinical trials in the United States. All of these current NA inhibitors were designed based upon the structure of 2-deoxy-2,3-didehydro- N -acetylneuraminic acid (Neu5Ac2en), a putative NA transition-state analogue [8] , [10] , [11] , [12] . Insight into the NA catalytic mechanism and the proposed oxocarbenium ion transition-state intermediate were crucial for the design of Neu5Ac2en analogues with potent NA inhibitory activity [13] , [14] . However, evidence regarding the key influenza NA catalytic residues has remained elusive and the successful design of highly effective next-generation influenza NA inhibitors has proven to be a difficult task. Influenza NA is a retaining glycosidase that cleaves the α-ketosidic bond of terminally linked sialic acid, notably N -acetylneuraminic acid (Neu5Ac), the predominant sialic acid in humans [8] . A majority of known retaining glycosidases utilize a pair of conserved active-site carboxylate residues with one functioning as a catalytic nucleophile in a double-displacement mechanism [15] , [16] . Retaining NA mechanisms, on the other hand, appear to be quite distinct. Biochemical analysis of NA from various microorganisms has revealed that a conserved active-site tyrosine can function as a nucleophile and may be the most important catalytic residue [17] , [18] , [19] . Although influenza NAs share very little sequence identity with NAs from other microorganisms, their active sites are highly conserved, which suggests that they all may function in a similar manner [8] . Leaving group effect and kinetic isotope effect experiments with influenza NA carried out by Guo et al. [16] and Chou et al. [20] are compatible with the classical mechanism that includes a covalent enzyme-sialosyl intermediate. Studies by Burmeister et al. [21] and Ghate et al. [22] also suggest that Tyr406 has an important role in the influenza NA mechanism. However, numerous studies still indicate that the influenza NA may possibly function in a unique manner. For example, 4-guanidino-Neu5Ac2en (zanamivir), 4-amino-Neu5Ac2en and even Neu5Ac2en all exhibit selectivity for influenza NA over NA from other species [10] ; a computational study by Thomas et al. [23] concluded that a direct hydroxylation mechanism with no covalent influenza NA-sialosyl intermediate is actually the energetically preferred pathway; moreover, some bacterial NAs that possess the same canonical protein fold and conserved active-site tyrosine still produce completely different products [16] , [24] . Taken together, the above studies clearly illustrate that the influenza virus NA catalytic mechanism may be quite unique. Therefore, experimental evidence is necessary to determine whether the influenza NA conserved active-site tyrosine is really a key catalytic residue and whether covalent inhibition of influenza NA is even possible. In this study, we first confirmed the catalytic role of the conserved active-site tyrosine (Tyr406, N2 numbering is used throughout the text) of influenza NA in order to explore the possibility of developing covalent influenza NA inhibitors. Influenza N2 was used as a classical example in this study, as N2-containing viruses are among the most common seasonal strains. Furthermore, the pathogenic agents of the 1957 H2N2 pandemic (Asian flu) and 1968 H3N2 pandemic (Hong Kong flu) are both N2-containing influenza A viruses. NMR and crystal soaking experiments clearly demonstrated that substitution of N2 Tyr406 with aspartic acid results in a switch of the influenza NA catalytic mechanism from a retaining glycosidase mechanism to an inverting mechanism. This further indicated that Tyr406 likely functions as a catalytic nucleophile; therefore, 2α,3ax-difluoro-Neu5Ac was synthesized and explored as a potential covalent influenza virus NA inhibitor. Soaking of N2 crystals with 2α,3ax-difluoro-Neu5Ac produced the first influenza virus NA covalent complex structure, proving that influenza NA Tyr406 functions as a catalytic nucleophile and that covalent NA inhibition is indeed possible. Most importantly, the covalent inhibitor 2α,3ax-difluoro-Neu5Ac achieved potent inhibition against both influenza A and B viruses as well as oseltamivir-resistant His274Tyr-NA. Tyr406 is the key catalytic residue of influenza NA Although Ghate et al. [22] were successful with the analysis of Tyr406Phe NA from influenza B 22 , a previous report by Lentz et al. [25] demonstrated that the phenylalanine 406 substitution actually results in an aberrantly processed influenza A N2 with loss of NA activity. Therefore, we chose a different approach by using a baculovirus expression system to produce recombinant N2 (rN2) from pandemic A/RI/5+/1957(H2N2) with a Tyr406Asp substitution. Substitution of Tyr406 with aspartic acid yielded a stable protein (rN2-Tyr406Asp) that was purified to homogeneity. 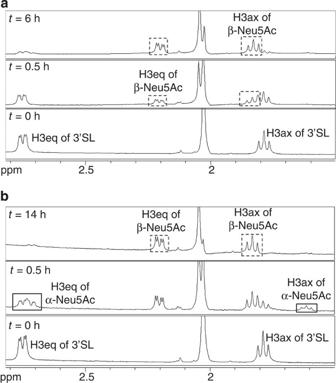Figure 1: Conserved Tyr406 is the key catalytic residue of influenza neuraminidase. (a)1H NMR analysis shows the initial and continuous production of β-Neu5Ac after incubation of rN2-Tyr406Asp with avian influenza receptor analogue 3′-sialyllactose, demonstrating that rN2-Tyr406Asp has shifted to an inverting glycosidase mechanism. (b) Wild-type influenza NA, in this case rN2, follows a retaining mechanism and therefore initially produces α-Neu5Ac from 3′-sialyllactose; the α-Neu5Ac undergoes mutarotation to form the more stable anomer, β-Neu5Ac, over time. rN2-Tyr406Asp had 100-fold reduced K cat and two-fold reduced K m as shown using kinetic analysis with a standard 4-methylumbelliferyl-Neu5Ac-based fluorescent assay ( Table 1 ). This confirms that Tyr406 is a critical factor for the catalytic activity of influenza NA. The enzymatic reaction of rN2 and rN2-Tyr406Asp was further monitored with 1 H NMR using the avian influenza receptor analogue 3′-sialyllactose. According to previous studies confirming that influenza NA is a retaining glycosidase [13] , wild-type rN2 initially produced α-Neu5Ac, which mutarotates to form the more stable β-Neu5Ac over time. Interestingly, the β-anomer of Neu5Ac was detected as the initial product of 3′-sialyllactose after incubation with rN2-Tyr406Asp, which demonstrates that rN2-Tyr406Asp has switched from a retaining to inverting glycosidase mechanism ( Fig. 1a and b ). Table 1 Fluorescence-based kinetic analysis of wild-type influenza rN2 compared with rN2-Tyr406Asp. Full size table Figure 1: Conserved Tyr406 is the key catalytic residue of influenza neuraminidase. ( a ) 1 H NMR analysis shows the initial and continuous production of β-Neu5Ac after incubation of rN2-Tyr406Asp with avian influenza receptor analogue 3′-sialyllactose, demonstrating that rN2-Tyr406Asp has shifted to an inverting glycosidase mechanism. ( b ) Wild-type influenza NA, in this case rN2, follows a retaining mechanism and therefore initially produces α-Neu5Ac from 3′-sialyllactose; the α-Neu5Ac undergoes mutarotation to form the more stable anomer, β-Neu5Ac, over time. Full size image A novel β-Neu5Ac-influenza NA complex structure rN2-Tyr406Asp was then crystallized and crystal soaking experiments were performed using 3′-sialyllactose. Despite its impaired catalytic activity, rN2-Tyr406Asp still hydrolysed the avian receptor analogue during soaking, resulting in the first influenza NA-β-Neu5Ac complex structure, at a resolution of 1.50 Å ( Fig. 2b ). 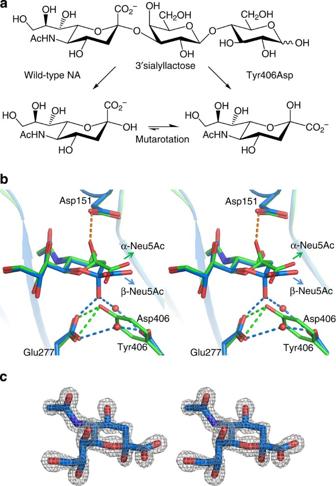Figure 2: N2-Tyr406Asp operates via an inverting sialidase mechanism. (a) Scheme outlining the initial formation of α-Neu5Ac by wild-type influenza NA and initial formation of β-Neu5Ac by influenza NA with a Tyr406Asp substitution. (b) Stereo illustration of the novel N2-Tyr406Asp-β-Neu5Ac complex (marine) in comparison to wild-type A/Tokyo/3/1967(H2N2) N2 complexed with α-Neu5Ac (green) (PDB ID: 2BAT). Two additional water molecules present in the N2-Tyr406Asp-β-Neu5Ac active site are coloured cyan. (c) Stereo illustration of β-Neu5Ac when bound to the N2-Tyr406Asp active site with the 2|Fo|-|Fc|map contoured at 2.0σ. Crystallographic data and refinement statistics are shown in Table 2 . Free sialic acids are much more stable in their β-anomeric configuration in solution; nevertheless, Neu5Ac always binds to wild-type NA as the α-anomer in a boat conformation [8] ( Fig. 2b ). The additional space created by substitution of Tyr406 with a smaller aspartic acid residue allows for the Neu5Ac to adopt a β-conformation where the C-2 hydroxy group in the N2-Tyr406Asp-β-Neu5Ac complex occupies the same region as the Tyr406 hydroxyl group of the wild-type complex. Furthermore, substitution of Tyr406 with Asp406 creates space for additional two water molecules between the C-2 hydroxyl group and Asp406 side-chain ( Fig. 2b ). Taken together, these results reveal that Tyr406 is indeed the key influenza NA catalytic residue and suggest that Tyr406 likely functions as a nucleophile that can be targeted by covalent inhibitors. Figure 2: N2-Tyr406Asp operates via an inverting sialidase mechanism. ( a ) Scheme outlining the initial formation of α-Neu5Ac by wild-type influenza NA and initial formation of β-Neu5Ac by influenza NA with a Tyr406Asp substitution. ( b ) Stereo illustration of the novel N2-Tyr406Asp-β-Neu5Ac complex (marine) in comparison to wild-type A/Tokyo/3/1967(H2N2) N2 complexed with α-Neu5Ac (green) (PDB ID: 2BAT). Two additional water molecules present in the N2-Tyr406Asp-β-Neu5Ac active site are coloured cyan. ( c ) Stereo illustration of β-Neu5Ac when bound to the N2-Tyr406Asp active site with the 2|Fo|-|Fc|map contoured at 2.0σ. Full size image Table 2 Crystallographic data collection and refinement statistics. Full size table Targeting influenza NA Tyr406 with a covalent inhibitor Based on our biochemical and structural analysis regarding the conserved Tyr406, we hypothesized that there was a high probability of targeting influenza virus NA with covalent inhibitors. In order for Tyr406 to undergo nucleophilic attack of the Neu5Ac anomeric carbon, a good leaving group should replace the C-2 hydroxyl group [26] . Another electronegative group at the C-3 position should also be present to destabilize any oxocarbenium ion transition-state intermediate, thereby stabilizing the potential Tyr406-inhibitor covalent bond [26] . Fluorinated compounds have been investigated for their anti-NA activity for quite some time and are excellent choices for covalent influenza NA inhibitors [26] , [27] , [28] , [29] , [30] . Although 2β,3eq-difluoro-Neu5Ac, which has been explored as an inhibitor of parainfluenza virus, was readily available from our previous studies [30] , structural analysis clearly demonstrates that the compound should be in the α-anomeric configuration so that the leaving group can face toward the outside of the NA active site cavity and depart easily ( Fig. 3a ). Therefore, 2α,3ax-difluoro-Neu5Ac was our primary target for a potential influenza virus NA covalent inhibitor. 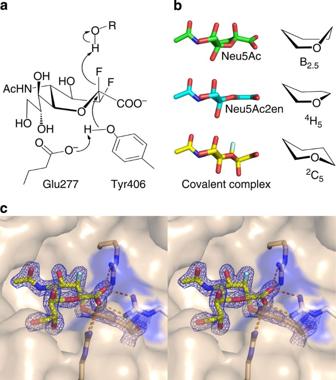Figure 3: Structure-based design and analysis of the first influenza NA covalent inhibitor. (a) Scheme for the mechanism-based design of covalent inhibition targeting influenza NA using 2α,3ax-difluoro-Neu5Ac. (b) Neu5Ac (green) adopts a boat conformation after binding to NA active site (PDB ID: 2BAT). Neu5Ac2en (cyan), a putative oxocarbenium ion transition state analogue, adopts a half-chair conformation(PDB ID: 1F8B). The covalently bound 3ax-fluoro-Neu5Ac moiety (yellow) adopts a chair conformation where C-2 moves toward Tyr406. This illustrates that in order to arrive at a covalently-linked intermediate, the reaction trajectory must still involve a planar intermediate. (c) Stereo illustration of the first influenza NA covalent complex, formed between rN2 Tyr406 (wheat) and a 3ax-fluoro-Neu5Ac moiety (yellow). The 2|Fo|-|Fc|map for the 3ax-fluoro-Neu5Ac moiety and Tyr406 is shown contoured at 2.0σ. Figure 3: Structure-based design and analysis of the first influenza NA covalent inhibitor. ( a ) Scheme for the mechanism-based design of covalent inhibition targeting influenza NA using 2α,3ax-difluoro-Neu5Ac. ( b ) Neu5Ac (green) adopts a boat conformation after binding to NA active site (PDB ID: 2BAT). Neu5Ac2en (cyan), a putative oxocarbenium ion transition state analogue, adopts a half-chair conformation(PDB ID: 1F8B). The covalently bound 3ax-fluoro-Neu5Ac moiety (yellow) adopts a chair conformation where C-2 moves toward Tyr406. This illustrates that in order to arrive at a covalently-linked intermediate, the reaction trajectory must still involve a planar intermediate. ( c ) Stereo illustration of the first influenza NA covalent complex, formed between rN2 Tyr406 (wheat) and a 3ax-fluoro-Neu5Ac moiety (yellow). The 2|Fo|-|Fc|map for the 3ax-fluoro-Neu5Ac moiety and Tyr406 is shown contoured at 2.0σ. Full size image 2α,3ax-difluoro-Neu5Ac is a potent influenza virus inhibitor 2α,3ax-difluoro-Neu5Ac indeed displayed potent in vitro NA inhibition, using both rN2 and live A/Jiangxi/262/2005(H3N2) virus, with IC 50 values of 201 and 286 nM, respectively ( Table 3 ). Inhibition of viral replication of seasonal A/Aichi/102/2008(H3N2) and A/Aichi/75/2008(H3N2) by 2α,3ax-difluoro-Neu5Ac in an AX4 cell-based assay was even more potent, both with IC 50 values of 16.1 nM ( Table 3 ). 2α,3ax-difluoro-Neu5Ac was also a highly potent low nanomolar level inhibitor of B/Lee/40 influenza B virus ( Table 3 , Fig. 4 ). Although no dramatic time dependent effects on influenza A virus NA inhibition were observed when using submicromolar concentrations of 2α,3ax-difluoro-Neu5Ac, inhibition of NA from B/Lee/40 resulted in more pronounced time-dependent effects, even at concentrations of 10–100 nM ( Fig. 4 ). Table 3 2α,3ax-difluoro-Neu5Ac is a potent inhibitor of influenza virus NA and influenza virus replication. 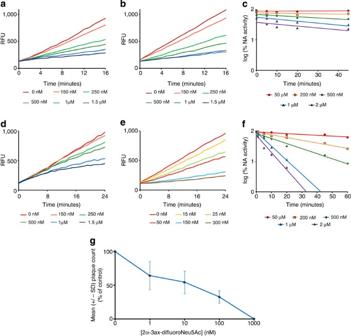Figure 4: Inhibition of A/Jiangxi/262/2005(H3N2) and B/Lee/40 influenza viruses. (a) Inhibition of A/Jiangxi/262/2005(H3N2) NA activity using no preincubation of virus with 0–1.5 μM 2α,3ax-difluoro-Neu5Ac (final concentration). (b) Inhibition of A/Jiangxi/262/2005(H3N2) NA activity using 30 min preincubation of virus with 0–1.5 μM 2α,3ax-difluoro-Neu5Ac (final concentration). (c) Plot of log[% H3N2 NA activity] versus incubation time for different preincubation concentrations of 2α,3ax-difluoro-Neu5Ac. (d) Inhibition of B/Lee/40 NA activity using no preincubation of virus with 0–1.5 μM 2α,3ax-difluoro-Neu5Ac (final concentration). (e) Inhibition of B/Lee/40 NA activity using 20 min preincubation of virus with 0–300 nM 2α,3ax-difluoro-Neu5Ac (final concentration). (f) Plot of log[% B/Lee/40 NA activity] versus incubation time for different preincubation concentrations of 2α,3ax-difluoro-Neu5Ac. (g) Inhibition of B/Lee/40 plaque formation by 1 nM, 10 nM, 100 nM and 1 μM 2α,3ax-difluoro-Neu5Ac. Each point with error bars represents the mean % plaque count (based upon 4 values for 1 nM and 6 values for 0 nM, 10 nM, 100 nM and μM)±s.d. Full size table Figure 4: Inhibition of A/Jiangxi/262/2005(H3N2) and B/Lee/40 influenza viruses. ( a ) Inhibition of A/Jiangxi/262/2005(H3N2) NA activity using no preincubation of virus with 0–1.5 μM 2α,3ax-difluoro-Neu5Ac (final concentration). ( b ) Inhibition of A/Jiangxi/262/2005(H3N2) NA activity using 30 min preincubation of virus with 0–1.5 μM 2α,3ax-difluoro-Neu5Ac (final concentration). ( c ) Plot of log[% H3N2 NA activity] versus incubation time for different preincubation concentrations of 2α,3ax-difluoro-Neu5Ac. ( d ) Inhibition of B/Lee/40 NA activity using no preincubation of virus with 0–1.5 μM 2α,3ax-difluoro-Neu5Ac (final concentration). ( e ) Inhibition of B/Lee/40 NA activity using 20 min preincubation of virus with 0–300 nM 2α,3ax-difluoro-Neu5Ac (final concentration). ( f ) Plot of log[% B/Lee/40 NA activity] versus incubation time for different preincubation concentrations of 2α,3ax-difluoro-Neu5Ac. ( g ) Inhibition of B/Lee/40 plaque formation by 1 nM, 10 nM, 100 nM and 1 μM 2α,3ax-difluoro-Neu5Ac. Each point with error bars represents the mean % plaque count (based upon 4 values for 1 nM and 6 values for 0 nM, 10 nM, 100 nM and μM)±s.d. Full size image In a previous mass spectrometric based analysis, binding of zanamivir and Neu5Ac2en to an 09N1 peptide containing Tyr406 was successfully detected [31] . Furthermore, covalent modification of the conserved active-site tyrosine was also detected in Trypanosoma rangeli sialidase using mass spectrometric methods [26] . Despite our attempts, we were unable to detect the covalent intermediate using similar methods; however, the observation of time-dependent inhibition indicates that the covalent intermediate is being formed in solution with influenza NA. One major concern for the use of fluorinated covalent inhibitors is toxicity; however, we observed no cytotoxity to MDCK cells when using up to 1 mM 2α,3ax-difluoro-Neu5Ac as determined by an MTT assay. Interestingly, 2β,3eq-difluoro-Neu5Ac was a better inhibitor of rN2-Tyr406Asp than wild-type rN2 (2 mM 2β,3eq-difluoro-Neu5Ac produced 54% inhibition of rN2-Tyr406Asp and only 25% inhibition of wild-type rN2). This can be explained by the rN2-Tyr406Asp-β-Neu5Ac complex structure, where the additional space resulting from the substitution of tyrosine with aspartic acid can better accommodate 2β,3eq-difluoro-Neu5Ac. The poor inhibition of rN2-Tyr406Asp by 2α,3ax-difluoro-Neu5Ac (>20 mM, Table 3 ) further indicated that it targets Tyr406 as a covalent inhibitor in solution. Probing the influenza virus NA covalent intermediate To determine if a covalent complex is really formed between influenza virus NA and 2α,3ax-difluoro-Neu5Ac, quality rN2 protein crystals were soaked with inhibitor and the complex crystal structure was solved at 1.80 Å. A N2-covalent complex structure was successfully obtained, with clear electron density revealing a 1.46 Å covalent bond between the Tyr406 terminal oxygen and the C-2 of a 3ax-fluoro-Neu5Ac moiety ( Fig. 3c ). The 3ax-fluoro-Neu5Ac moiety carboxylate is shifted closer toward Arg118 and away from Arg292 relative to N2 complexed with Neu5Ac. As expected, the C-2 fluoride leaving group is not present, confirming that it has departed during the formation of the molecular bond with Tyr406. Although no method is readily available to directly detect a naturally occurring covalent NA intermediate, the ability to obtain the influenza NA covalent complex using 2α,3ax-difluoro-Neu5Ac still suggests that a covalently bound intermediate is a critical step during hydrolysis of natural NA substrates. Therefore, we propose that influenza NA follows a double-displacement mechanism similar to the classical retaining glycosidase mechanism [16] . The covalently linked 3ax-fluoro-Neu5Ac moiety adopts a chair conformation, whereas α-Neu5Ac and Neu5Ac2en adopt boat and half-chair conformations [10] , respectively, when bound to influenza NA ( Fig.3b ). In our N2-covalent complex, the unique C-3 fluorine of the 3ax-fluoro-Neu5Ac moiety is 3.51–3.55 Å away from the closest neighbouring residue Arg118. Aside from the differences regarding C-2 due to a novel covalent bond and chair conformation, the remaining interactions between the 3ax-fluoro-Neu5Ac moiety and influenza NA highly resemble those of α-Neu5Ac and Neu5Ac2en. Effective covalent inhibition of oseltamivir-resistant NA The similarity of the 3ax-fluoro-Neu5Ac moiety binding mode to the natural NA ligand Neu5Ac is a strong indication that the covalent inhibitor 2α,3ax-difluoro-Neu5Ac should be effective against drug-resistant NA. This is also illustrated by the high similarity between the binding modes of the covalent inhibitor and zanamivir, which remain effective against oseltamivir-resistant His274Tyr NA [32] ( Fig. 5 ). Therefore, we also tested inhibition against oseltamivir-resistant rN1-His274Tyr from the 2009 H1N1 pandemic in comparison to wild-type rN1. Although His274Tyr N1 has been reported to exhibit more than 200-times lower inhibition by oseltamivir than by wild-type N1 [32] , the covalent inhibitor 2α,3ax-difluoro-Neu5Ac inhibited recombinant 2009 pandemic N1 (r09N1-His274Tyr) at the same level as wild-type recombinant 2009 pandemic N1 (r09N1) ( Table 3 ). This demonstrates that 2α,3ax-difluoro-Neu5Ac is an effective inhibitor against the most common oseltamivir-resistant NA. 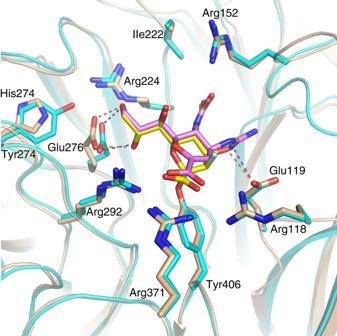Figure 5: Structural comparison of the N2-covalent complex with the oseltamivir-resistant N1-His274Tyr zanamivir complex. The binding mode of the 3ax-fluoro-Neu5Ac moiety (yellow) in N2 (wheat) and zanamivir (violet) in N1-His274Tyr (cyan) (PDB ID: 3CKZ) is highly similar, indicating that 2α,3ax-difluoro-Neu5Ac should remain effective against common oseltamivir-resistant influenza viruses. Figure 5: Structural comparison of the N2-covalent complex with the oseltamivir-resistant N1-His274Tyr zanamivir complex. The binding mode of the 3ax-fluoro-Neu5Ac moiety (yellow) in N2 (wheat) and zanamivir (violet) in N1-His274Tyr (cyan) (PDB ID: 3CKZ) is highly similar, indicating that 2α,3ax-difluoro-Neu5Ac should remain effective against common oseltamivir-resistant influenza viruses. Full size image In this study, we confirm that the conserved active site Tyr406 has an integral role in the catalytic mechanism of influenza virus NA and that Tyr406 can be successfully targeted for the design of covalent inhibitors. Furthermore, due to its importance in the catalytic cycle, drug-resistant mutations leading to substitution of Tyr406 are extremely unfavourable for the influenza virus. This is further illustrated by the fact that Tyr406 is almost 100% conserved among all influenza virus NA proteins. Therefore, the targeting of Tyr406 with covalent inhibitors is a next-generation strategy for influenza inhibitor development, which is highly advantageous in terms of drug resistance. However, the first generation of influenza NA competitive inhibitors are still highly vulnerable to drug resistance. Long before the widespread circulation of natural oseltamivir-resistant influenza virus strains, it had been proposed that inhibitors that more closely resemble natural NA ligands are less likely to develop drug resistance [33] . Oseltamivir contains a hydrophobic pentyl ether group in place of the glycerol moiety of the natural NA ligand Neu5Ac and therefore oseltamivir resistance is easily developed. Upon binding of natural NA ligands, Glu276 hydrogen bonds with the ligand glycerol moiety. However, in order to accommodate oseltamivir, Glu276 must rotate to form a salt bridge with Arg224. The most common oseltamivir-resistant mutations, like His274Tyr, interfere with the rotation of Glu276, which is necessary to accommodate oseltamivir [32] . Although zanamivir resistance is not as common as oseltamivir resistance due to a higher similarity with Neu5Ac, amino-acid substitutions, like Glu136Lys, can still arise that interfere with the binding of the zanamivir C-4 guanidino group. Aside from the similarity with the natural NA ligand, Neu5Ac, zanamivir is also not as commonly used as oseltamivir, which contributes to the lower frequency of zanamivir-resistant viruses. Nevertheless, the oseltamivir hydrophobic pentyl ether and the zanamivir C-4 guanidino that contribute to drug resistance are the key modifications that contribute to their potency. Therefore, 2α,3ax-difluoro-Neu5Ac, which more closely resembles the natural NA ligand, can still exhibit highly potent inhibition due to its action as a covalent inhibitor, and thus possesses significant advantages. Still, rational modification of 2α,3ax-difluoro-Neu5Ac should be vigorously pursued to produce more potent next-generation covalent influenza virus NA inhibitors. As we observe stronger time-dependent inhibition ( Fig. 4 ) in combination with a significant increase in potency ( Table 3 ) for influenza B NA, the increased time dependence must be a result of an increased lifetime of a reversible covalent intermediate rather than an effect of slow inhibitor binding [34] . Therefore, this illustrates that further stabilization of the covalent intermediate is a promising strategy to improve the effectiveness of next-generation covalent influenza virus NA inhibitors. Two major strategies can be taken for the stabilization of the influenza NA Tyr406-inhibitor covalent bond: modification of the covalent inhibitor to disrupt steric effects imposed by the NA active site that destabilize the favored chair conformation of the covalent intermediate, and modification of the covalent inhibitor to further destabilize build-up of positive charge around C-2, thereby stabilizing the covalent intermediate. In regards to the first strategy, it is difficult to predict from our complex structure, what specific modifications will stabilize the chair conformation of the covalent intermediate. In regards to the second strategy, a stronger C-3 electron-withdrawing group might increase the lifetime of the covalent intermediate. As observed in the N2-covalent complex structure, there is no significant interaction between the 3-ax-fluoro-Neu5Ac moiety 3-ax-fluorine with influenza N2, indicating that the C-3 fluorine contributes to the inhibition potency by stabilization of the covalent intermediate. The lack of interactions between the 3-ax-fluorine and the NA active site should also allow for sufficient room to accommodate a bulkier, stronger C-3 electron-withdrawing group that may further stabilize the NA covalent intermediate. Although the closed conformation of the 150-loop in group 2 NA structures as well as the 2009 pandemic N1 [40] could potentially hinder the binding of a bulkier C-3 group, recent studies have demonstrated that the 150-loop is inherently flexible [35] and, therefore, is able to accommodate bulkier electron-withdrawing groups. In conclusion, this study contributes the first proof-of-concept for the use of covalent influenza NA inhibitors as a true next-generation strategy for influenza drug development. The first-generation influenza NA inhibitors, zanamivir and oseltamivir, are regarded as a classical example of structure-based competitive inhibitor design; however, novel strategies for NA inhibition has remained limited. The first covalent influenza NA-complex offered here provides a framework for the rational and structure-based development of highly potent next-generation influenza virus inhibitors of the future. Cells and viruses AX4 cells, MDCK cells with increased levels of sialyl-α2,6-galactose moieties, were grown and maintained following previous protocols [36] , [37] . The seasonal influenza virus isolates A/Aichi/102/2008(H3N2), A/Aichi/75/2008(H3N2) (Aichi Pref. Inst. Public Health, Japan), A/Jiangxi/262/2005(H3N2) (China CDC) and recombinant B/Lee/40 were amplified in MDCK cells. Viral culture supernatants were harvested, concentrated and stored at −80 °C. Expression and purification of influenza NAs Recombinant NAs were purified to homogeneity after being expressed in a baculovirus expression system, based on the original method by Xu et al. [38] , [39] , [40] , [41] with modifications. For rN2-Tyr406Asp and 2009 pandemic rN1-His274Tyr, point mutations were introduced by site-directed mutagenesis based upon the corresponding wild-type NAs (Generay, China). Enzymatic kinetics The activity of rN2 and rN2-Tyr406Asp was monitored using a fluorometric assay based on methods from Potier et al. [42] NA activity was monitored using 0–500 μM 4-methylumbelliferyl-Neu5Ac (J&K Scientific) with 33 mM MES and 4 mM CaCl 2 (pH 6.0). The final concentration of enzymes used for wild-type rN2 and rN2-Tyr406Asp were 1 and 167 nM, respectively. Reactions were performed in a total volume of 50 μl at 37 °C, and monitored every 30 s over the course of 30 min on a SpectraMax M5 (Molecular Devices) at excitation and emission wavelengths of 355 and 460 nm, respectively. All assays were performed in no less than triplicates and the final data were fitted to the Michaelis–Menten equation using GraphPad Prism to determine the Michaelis–Menten constant ( K m ) and maximum velocity of substrate conversion ( V max ). In vitro NA inhibition assay A 4-methylumbelliferyl-Neu5Ac-based fluorometric NA assay was also used to test competitive NA inhibition [42] . Recombinant NA or live influenza virus was diluted until NA activity was in the appropriate range for fluorescence detection of liberated 4-methylumbelliferone on a SpectraMax M5 (Molecular Devices), using excitation and emission wavelengths of 355 and 460 nm, respectively. 4-methylumbelliferyl-Neu5Ac was used at a final concentration of 100 μM. Five concentrations of 0–5 μM 2α,3ax-difluoro-Neu5Ac and a positive control with an equivalent volume of PBS were used for each replicate. For quantification of the B/Lee/40 half maximal inhibitory concentration (IC 50 ), 2α,3ax-difluoro-Neu5Ac was preincubated with live B/Lee/40 virus for 20 min before starting the reaction. For influenza A NA, all components were mixed simultaneously at the start of the reaction. Each assay was done in no less than triplicates. IC 50 values were determined by plotting log[inhibitor] versus per cent inhibition using the sigmoidal dose response (variable slope) function in GraphPad Prism. 1 H NMR NA activity assay 1 H NMR spectroscopy (600 MHz Bruker DXM-600, Bruker, CAS Institute of Biophysics) was employed to monitor the hydrolysis of 3′-sialyllactose (Carbosynth) catalysed by NA until the reactions reached equilibrium. For each reaction, a total volume of 500 μl with the ratio of D 2 O to H 2 O of 1:9 was used, containing enzyme, 2 mM substrate, 20 mM phosphate, 100 mM NaCl and 1 mM CaCl 2 (pH 6.0). The final concentrations for wild-type rN2 and rN2-Tyr406Asp were 32 nM and 13 μM, respectively. Spectral data were collected at 37 °C with 64 scans and a relaxation delay of 2 s. An initial spectrum containing only substrate and buffer (without NA) was acquired and referred to as time zero. The same reactions were also performed at 25 °C for monitoring and no obvious difference was seen. Crystallization, soaking and data collection The baculovirus expression system allows for the production of high quantities of soluble NA for crystallization experiments; however, despite our recent success with the structural characterization of 09N1 (ref. 40 ), we were unable to obtain enough quality N1 crystals for the soaking experiments carried out in this study. Instead, quality rN2 crystals were obtained as previously described [41] , and rN2-Tyr406Asp crystals were grown by vapour diffusion in hanging drops that consist of 1 μl concentrated protein (6 mg ml −1 ) and 1 μl reservoir solution (0.1 M MES monohydrate pH 6.0, 14% w/v polyethylene glycol 4000). rN2 and rN2-Tyr406Asp crystals were soaked in the corresponding mother liquor containing 10 mM of 2α,3ax-difluoro-Neu5Ac2 at 4 °C for 45 min and 10 mM 3′-sialyllactose at 18 °C for 180 min, respectively. After flash-cooling at 100 K with cryoprotection, diffraction data were collected at SSRF beamline BL17U and KEK beamline BL17A for the N2-Tyr406Asp-β-Neu5Ac complex and N2-covalent complex, respectively. Data processing and structure solution Diffraction data were processed and scaled using HKL2000 (ref. 43 ) and the statistics are outlined in Table 2 . The structure of N2-Tyr406Asp complexed with β-Neu5Ac and the wild-type N2-covalent complex were both determined by molecular replacement using Phaser [44] from the CCP4 suite [45] with the structure of A/Tokyo/3/1967(H2N2)N2 (PDB ID: 1IVG) as the search model. REFMAC5 (ref. 46 ) and COOT [47] were employed for initial restrained rigid-body refinement and model building, respectively. Further cycles of refinement were carried out with phenix.refine implemented in the Phenix package [48] . The stereochemical quality of the obtained model was finally assessed using Procheck [49] . Cytotoxicity assay Cytotoxicity was assessed in MDCK cells following a standard MTT assay protocol [50] . AX4 cell-based virus inhibition assay Inhibition of influenza virus propagation was measured using AX4 cells in the presence of serial dilutions of 2α,3ax-difluoro-Neu5Ac (0.1–100 μM) [37] , [51] . Influenza virus at a multiplicity of infection of 0.03 was preincubated with a medium containing 2 μg ml −1 acetylated trypsin in the absence or presence of serially diluted inhibitor for 1 h at 4 °C. Then, the inhibitor–virus mixture was added onto the AX4 cell monolayers, which were incubated for 18–20 h at 37 °C. Infected cells were fixed and permealized with methanol followed by staining with antiviral NP mouse antibody and β-galactosidase-conjugated anti-mouse IgG. A substrate solution containing 4-methylumbelliferyl-β- D -galactoside and MgCl 2 was added to initiate the galactosidase reaction. 4-methylumbelliferyl was detected with an excitation wavelength of 355 nm and an emission wavelength of 460 nm on a Mithras LB940 microplate reader (Berthold Technologies, Pforzheim, Germany) to determine the virus titre in the infected cells. The infectious foci were also observed using a peroxidase-based chromogenic assay. The cells were treated with HRP-conjugated goat anti-mouse IgG antibody and influenza virus was stained blue by incubation with H 2 O 2 , N,N -diethyl- p -phenylenediamine dihydrochloride and 4-chloro-1-naphthol. EC 50 values were calculated graphically with GraphPad Prism using the fluorescent assay data. Eleven replicates were used for A/Aichi/102/2008 H3N2 and six replicates were used for A/Aichi/75/2008 H3N2. Plaque-reduction assay The effectiveness of 2α,3ax-difluoro- N -acetylneuraminic acid against influenza plaque reduction was assessed with recombinant B/Lee/40 influenza virus based on a previously reported method [52] . MDCK cell monolayers were inoculated with virus ( ∼ 40 PFU per well) and the plates were incubated for 1 h at 37 °C. The inoculum was then removed and an agarose overlay containing appropriate inhibitor dilution was added. After 2 days of incubation at 37 °C, the results of plaques reduction were recorded, and the EC 50 values were calculated graphically using GraphPad Prism. Six replicates were used for the plaque-reduction assay. How to cite this article: Vavricka, C.J. et al. Influenza neuraminidase operates via a nucleophilic mechanism and can be targeted by covalent inhibitors. Nat. Commun. 4:1469 doi: 10.1038/ncomms2487 (2013).